Cobalt-catalyzed electrooxidative C-H/N-H [4+2] annulation with ethylene or ethyne Ethylene and ethyne are among the simplest two-carbon building blocks. However, quite limited methods can be applied to incorporate ethylene or ethyne into fine chemicals. Here we demonstrate a cobalt-catalyzed dehydrogenative C–H/N–H [4+2] annulation of aryl/vinyl amides with ethylene or ethyne by using an electrochemical reaction protocol. Significantly, this work shows an example of electrochemical recycling of cobalt catalyst in oxidative C–H functionalization reactions, avoiding the use of external chemical oxidants and co-oxidants. The electrochemical method provides a reliable and safe way for incorporating gas-phase ethylene or ethyne into fine chemicals. High reaction efficiency and good functional group tolerance are observed under divided electrolytic conditions. Ethylene is the most abundantly produced organic molecule by volume in petroleum industry [1] , [2] . A large amount of ethyne can be easily obtained by the partial combustion of methane [3] . Both ethylene and ethyne represent the simplest, readily functionalized, and inexpensive two-carbon synthons in organic chemistry. However, quite a limited number of methods have been reported to directly incorporate ethylene or ethyne into fine chemicals [4] . This might be partially due to the apprehensions about operating with gas-phase reactants, especially under oxidative conditions. Admittedly, the mixture of ethylene or ethyne with oxygen is quite dangerous since it can easily cause explosion. Thus, it is of great challenge to apply ethylene and ethyne as standard substrates in oxidative cross-coupling reactions. Over the past decade, transition metal catalyzed oxidative C–H functionalization has been developed as an efficient and atom-economical method for the direct cross-coupling of arenes with alkenes and akynes [5] , [6] , [7] . However, most of these methods are only able to apply substituted alkenes or alkynes as the substrates [8] . Moreover, external chemical oxidants are generally required for the recycling of the metal catalysts, which inevitably brings undesired oxidation byproducts. In 2007, Jutand and co-workers [9] described an electrochemical oxidation promoted dehydrogenative Heck reaction between N -acetylanilines and alkenes. Pd(OAc) 2 was used as the key catalyst while 1,4-benzoquinone was added as a co-catalyst. During the reaction process, 1,4-benzoquinone acted as a redox mediator for oxidizing Pd(0) to Pd(II) by anode. Though with a limited substrate scope and low reaction efficiency, this work demonstrated the first example of electrochemical recycling of palladium catalyst in oxidative C–H functionalization reactions. During the following years, electrochemical oxidation has also been used in other palladium-catalyzed oxidative C–H functionalization reactions [10] , [11] , [12] , [13] . However, the electrochemical recycling of other transition metal catalysts in oxidative C–H functionalization has rarely been developed [14] , [15] . Owing to the low costs and low toxicity of cobalt salts, cobalt-catalyzed C–H functionalization has attracted increasing attentions over the past few years [16] , [17] , [18] . As for oxidative C–H functionalization, the stoichiometric amount of high-valent metal salts especially silver salts and manganese salts are generally required to recycle the cobalt catalysts [19] , [20] , [21] , [22] , [23] , [24] , [25] , [26] . In 2014, Daugulis and co-workers [27] , [28] first reported the cobalt-catalyzed oxidative C–H/N–H [4+2] annulation with alkynes and alkenes. In their reaction system, the stoichiometric amount of manganese salt was required for the reaction with alkyne and half an equivalent of manganese salt was essential for the reaction with alkene. More significantly, the use of oxygen as the terminal oxidant limits its potential application to incorporate ethylene and ethyne into fine chemicals due to the safety issues. Here we demonstrate a cobalt-catalyzed electrooxidative C–H/N–H [4+2] annulation between aryl/vinyl amides and ethylene/ethyne. Cobalt catalyst is directly recycled by anodic oxidation under external oxidant-free conditions. During the submission of this manuscript, Ackermann and co-workers [29] reported a cobalt-catalyzed electrooxidative C–H/N–H [4+2] annulation between aryl/vinyl amides and terminal alkynes. Investigation of reaction conditions N -(quinolin-8-yl)benzamide ( 1a ) was chosen as the model substrate to test the reaction conditions. After considerable efforts, dehydrogenative C–H/N–H [4+2] annulation with ethylene was successfully achieved by using Co(acac) 2 as the catalyst in the presence of sodium pivalate under divided electrolytic conditions. 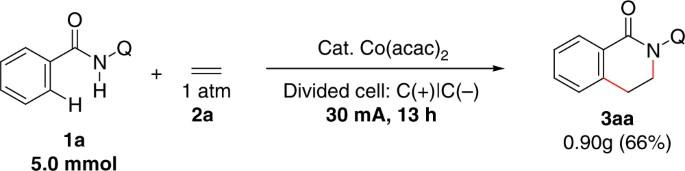Fig. 1 Large-scale synthesis. Gram scale reaction with ethylene under electrochemical conditions Eighty-nine percent isolated yield of the cyclization product 3aa could be obtained at 4.0 mA constant current electrolysis after 4 h (Table 1 , entry 1). It is worthy of noting that the aminoquinoline directing group was essential for this electrochemical reaction since no desired product could be observed by using pyridine or pyridine- N -oxide as the directing group. The choice of a cobalt catalyst precursor was important for obtaining a high reaction yield. Replacing Co(acac) 2 by CoCl 2 or Co(OAc) 2 led to decreased product yields (Table 1 , entries 2 and 3). The additive was also beneficial for achieving a good reaction efficiency. Only trace amount of the desired product could be detected in the absence of NaOPiv·H 2 O or using CF 3 SO 3 Na instead of NaOPiv·H 2 O (Table 1 , entries 4 and 5). Applying HCOONa·H 2 O instead of NaOPiv·H 2 O led to a low reaction yield (Table 1 , entry 6). Seventy-two percent yield could be obtained with NaOAc (Table 1, entry 7) while 85% yield could be obtained with PhCOONa·H 2 O (Table 1 , entry 8). 2,2,2-Trifluoroethanol was found to be the most efficient solvent in this transformation while acetonitrile or ethanol gave dramatically decreased reaction yields (Table 1 , entries 9 and 10). As for the selection of electrode material, a platinum plate cathode and a carbon cloth cathode showed similar reactivity with a nickel plate cathode (Table 1 , entries 11 and 12). However, the platinum plate was not so efficient when it was used as the anode material instead of the carbon cloth anode (Table 1 , entry 13). No desired product could be observed without electric current (Table 1 , entry 14). Nevertheless, the operating electric current did not exert much influence on the reaction efficiency. Slightly decreased reaction yields could still be obtained either by increasing or decreasing the operating current (Table 1 , entries 15 and 16). The result observed by increasing operating current provides possibilities for larger scale synthesis. We have tried to do a 5 mmol scale reaction in a larger divided cell with 30 mA constant current. Carbon cloth was used as the electrode material for both anode and cathode. Delightfully, 0.90 g (66%) of 3a could be obtained after 13 h electrolysis (Fig. 1 ). Table 1 Effects of the reaction parameters Full size table Fig. 1 Large-scale synthesis. Gram scale reaction with ethylene under electrochemical conditions Full size image Substrate scope The scope of amides in this dehydrogenative annulation reaction was in turn explored (Fig. 2 ). Benzamides bearing one ortho methyl group or two meta methyl groups all showed similar reactivity with simple benzamide ( 3aa-3ca ). Notably, bromide substituent at the para position was well tolerated, which provides possibility for further functionalization ( 3da ). Amides bearing the electron-donating group or the electron-withdrawing group at the para position all showed good reaction efficiency in this transformation ( 3ea and 3fa ). Besides benzamides, other aromatic amides such as thiophene-2-carboxamide and furan-2-carboxamide were able to furnish the desired products in good yields ( 3ga and 3ha ). Significantly, vinyl amides were also suitable substrates in this electrooxidative [4+2] annulation reaction. Methacrylamide and cinnamamide could react with ethylene to afford the desired annulation products in moderate yields ( 3ia and 3ja ). Notably, tri-substituted vinyl amide could give the annulation product in 80% yield ( 3ka ). Fig. 2 Electrooxidative C–H/N–H [4+2] annulation with ethylene. Reaction conditions: 1 (0.20 mmol), Co(acac) 2 (15 mol%), NaOPiv·H 2 O (1.5 equiv), n Bu 4 NBF 4 (3.0 equiv), CF 3 CH 2 OH (8.0 mL) [anode], and NaOPiv·H 2 O (1.5 equiv), HOPiv (10 equiv), MeOH (8.0 mL) [cathode] in and H-type divided cell with carbon cloth anode, nickel plate cathode, and an AMI-7001-30 membrane, constant current = 4.0 mA ( J anode = 1.8 mA/cm 2 ), ethylene balloon (1 atm), 70 °C, 4 h (3.0 F/mol). Isolated yields are shown Full size image Under the similar reaction conditions as ethylene, ethyne was also found to be a suitable two carbon linker in this dehydrogenative C–H/N–H [4+2] annulation (Fig. 3 ). Besides, similar functional group tolerance was observed for aryl amides ( 3ab ). Benzamides bearing ortho and meta methyl groups showed good reactivity in this transformation ( 3bb and 3cb ). Para -bromo benzamide was still a suitable substrate though with a decreased reaction yield ( 3db ). Both electron-rich and electron-deficient benzamides could afford the desired products in high yields ( 3eb and 3fb ). Thiophene-2-carboxamide and furan-2-carboxamide could also react with ethyne to give the desired aromatic compounds ( 3gb and 3hb ). Similar to the study with ethylene, vinyl amides were also tested as substrates. Methacrylamide reacted with ethyne with 49% yield ( 3ib ) while cinnamamide could provide a 79% yield ( 3jb ). Tri-substituted vinyl amide also furnished an annulation product in 76% yield ( 3kb ). Besides the reaction with ethylene and ethyne, substituted alkenes and alkynes were also suitable in the electrochemical [4+2] annulation reaction. Selected examples are shown in Supplementary Fig. 3 . Fig. 3 Electrooxidative C–H/N–H [4+2] annulation with ethyne. Reaction conditions: 1 (0.20 mmol), Co(acac) 2 (10 mol%), NaOPiv·H 2 O (2 equiv), n Bu 4 NBF 4 (3.0 equiv), CF 3 CH 2 OH (8.0 mL) [anode], and NaOPiv·H 2 O (2.0 equiv), HOPiv (10 equiv), MeOH (8.0 mL) [cathode] in and H-type divided cell with carbon cloth anode, nickel plate cathode, and an AMI-7001-30 membrane, constant current = 5.0 mA ( J anode = 2.2 mA/cm 2 ), ethyne balloon (1 atm), 70 °C, 3 h (2.8 F/mol). Isolated yields are shown Full size image In the next step, experiments were carried out to get some insights into the reaction mechanism. First, kinetic isotope experiments were performed to probe the C–H activation step. An intermolecular competition experiment between 1a and [D 5 ] - 1a was done. The ratio of the [4+2] oxidative annulation products 3aa and [D 4 ]-3aa was determined as 3.5:1 (Fig. 4a ). Parallel reactions of 1a and [D 5 ]-1a were carried out and the reaction rates were determined separately, giving a KIE value of 1.4 (Fig. 4b , k H / k D ). Since only secondary isotope effect was observed in the parallel reactions, the C–H bond cleavage was a slow step but not likely to be the rate-determining step [30] . Fig. 4 Kinetic isotope effect experiments. a Intermolecular competition experiment between 1a and [D 5 ]-1a . b Parallel reactions with 1a and [D 5 ]-1a Full size image Preliminary kinetic studies were also carried out to determine the order of reaction components for the cobalt-catalyzed electrooxidative C–H/N–H [4+2] annulation between 1a and ethylene. It is worthy of noting that induction period was observed in most of the reactions. The initial reaction rates were monitored by GC analysis upon changing the concentration of 1a , NaOPiv·H 2 O, and cobalt catalyst. The reaction rates were almost invariant under different concentrations of 1a or NaOPiv·H 2 O (Fig. 5a, b ). Thus, substrate binding or deprotonation might not be involved in the rate-determining step. Interestingly, the reaction rate was even independent on the concentration of Co(acac) 2 (Fig. 5c ) while the initial reaction rates changed with different operating currents (Fig. 5d ). These results suggested that the electrochemical oxidation was likely to be the rate-limiting step during electrolysis. Fig. 5 Kinetic studies for the cobalt-catalyzed electrooxidative C–H/N–H [4+2] annulation between 1a and ethylene. a Kinetic profiles under different concentrations of 1a . b Kinetic profiles under different concentrations of NaOPiv·H 2 O. c Kinetic profiles under different concentrations of Co(acac) 2 . d Kinetic profiles under different operating currents Full size image After that, we studied the electrochemical oxidation step by performing cyclic voltammetry (CV) experiments. An obvious oxidation peak of substrate 1a could be observed at 1.47 V (Fig. 6a , blue line). As for Co(acac) 2 , two relatively weak oxidation peaks were observed at 1.12 and 1.53 V (Fig. 6a , red line). These results indicated that Co(II) species was probably oxidized by anode before 1a . Moreover, the mixture of Co(acac) 2 and 1a demonstrated a stronger oxidation peak at 1.13V when compared with the oxidation peaks only observed with Co(acac) 2 (Fig. 6a , green line). According to our previous EXAFS study on the oxidation of Co(acac) 2 by Ag 2 CO 3 [31] , Co(III) species were likely to be generated through the anodic oxidation of the coordinated Co(II) species. During current controlled electrolysis, the working voltage for whole electrolytic cell ranged from 7.50 to 8.50 V while the oxidation potential of anode (vs Ag/AgCl) ranged from 1.24 to 1.60 V. To confirm the assumption that coordinated Co(II) species were the key intermediate in electrochemical oxidation, the reaction was conducted at the first peak oxidation potential of the mixture of Co(acac) 2 and 1a . Notably, the potential controlled electrolysis at 1.13 V afforded 3aa in 70% yield (Fig. 6b ). Fig. 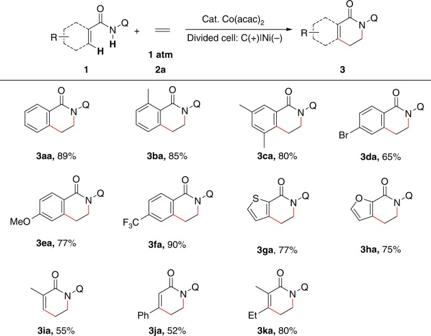Fig. 2 Electrooxidative C–H/N–H [4+2] annulation with ethylene. Reaction conditions:1(0.20 mmol), Co(acac)2(15 mol%), NaOPiv·H2O (1.5 equiv),nBu4NBF4(3.0 equiv), CF3CH2OH (8.0 mL) [anode], and NaOPiv·H2O (1.5 equiv), HOPiv (10 equiv), MeOH (8.0 mL) [cathode] in and H-type divided cell with carbon cloth anode, nickel plate cathode, and an AMI-7001-30 membrane, constant current = 4.0 mA (Janode= 1.8 mA/cm2), ethylene balloon (1 atm), 70 °C, 4 h (3.0 F/mol). Isolated yields are shown 6 Study of the oxidation potential during the electrolysis. a Cyclic voltammograms in CF 3 CH 2 OH (10 mL) with 0.06 M n Bu 4 NBF 4 : blue line, 1a (0.050 mmol); red line, Co(acac) 2 (0.050 mmol); green line, a mixture of Co(acac) 2 (0.050 mmol), and 1a (0.050 mmol). b Potential controlled electrolysis at 1.13 V (vs Ag/AgCl) Full size image Based on the above-mentioned results, a possible mechanism for this cobalt-catalyzed electrooxidative C–H/N–H annulation reaction between 1a and ethylene is proposed in Fig. 7 . Initially, Co(II) complex coordinates with 1a , with the help of NaOPiv·H 2 O affording a bidentate nitrogen coordinated Co(II) complex A . Next, complex A is directly oxidized by anode to afford Co(III) complex B . With the assistance of NaOPiv·H 2 O, intramolecular C−H activation of complex B takes place to generate a cyclic Co(III) complex C . Then, ethylene ( 2a ) insertion and reductive elimination of the Co(III) species form the final product 3aa . Finally, the Co(I) species generated after reductive elimination are oxidized by carbon anode to regenerate the Co(II) catalyst. Proton reduction is likely to be the concomitant cathodic reaction since a large amount of hydrogen gas can be detected by GC in the reaction system after the reaction is stopped. Fig. 7 Proposed mechanism for the reaction between 1a and 2a . Tentative reaction mechanism involves anodic oxidation of the coordinated Co(II) complex to generate a Co(III) complex, intramolecular C−H activation, ethylene insertion, and reductive elimination of Co(III) species to form the annulation product, and finally a second anodic oxidation to regenerate the Co(II) catalyst Full size image In conclusion, we have demonstrated an example of recycling the cobalt catalyst by electrochemical anodic oxidation in oxidative C–H functionalization reactions. This electrochemical reaction protocol enables the dehydrogenative C–H/N–H annulation with ethylene or ethyne under external oxidant-free conditions. The reaction exhibits high functional group tolerance. Both aryl and vinyl amides are suitable substrates in this transformation, which affords the desired [4+2] annulation products in good to high reaction yields. Preliminary mechanistic study indicates that electrochemical oxidation of coordinated Co(II) complex may be the key step during the reaction process. The study of recycling other transition metals by anodic oxidation in oxidative C–H functionalization reactions is underway in our laboratory. Electrooxidative C–H/N–H [4+2] annulation with ethylene (Method A) The electrolysis was carried out in an oven-dried H-type divided cell equipped with two stir bars. Carbon cloth (15 mm × 15 mm × 0.36 mm) was used as the anode and the nickel plate (15 mm×15 mm×1.0 mm) was used as the cathode. The two electrodes were separated by an ULTREX ® AMI-7001-30 membrane. The anodic chamber was added with amide (0.20 mmol), Co(acac) 2 (0.030 mmol, 7.7 mg), NaOPiv·H 2 O (0.30 mmol, 42.6 mg), and n Bu 4 NBF 4 (0.60 mmol, 197.6 mg) while the cathodic chamber was added with NaOPiv·H 2 O (0.30 mmol, 42.6 mg) and HOPiv (2.0 mmol, 204.3 mg). A balloon filled with ethylene (1 atm) was connected to the electrolysis system and purged for three times. Subsequently, CF 3 CH 2 OH (8.0 mL) and MeOH (8.0 mL) were added to the anodic chamber and cathodic chamber respectively. Then the electrolysis system was stirred at a constant current of 4.0 mA at 70 °C for 4 h. When the reaction was finished, the reaction mixture of the anodic chamber was washed with water and extracted with diethyl ether (10 mL × 3). The organic layers were combined, dried over Na 2 SO 4 , and concentrated. The pure product was obtained by flash column chromatography on silica gel (petroleum: ethyl acetate = 1:1). Full experimental details and characterization of the compounds are given in the Supplementary Information. 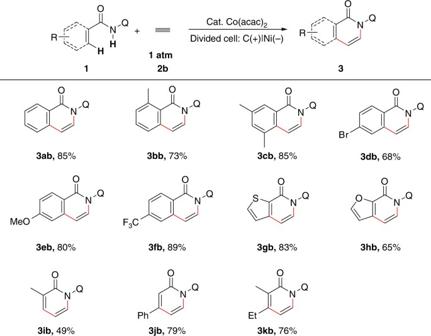Fig. 3 Electrooxidative C–H/N–H [4+2] annulation with ethyne. Reaction conditions:1(0.20 mmol), Co(acac)2(10 mol%), NaOPiv·H2O (2 equiv),nBu4NBF4(3.0 equiv), CF3CH2OH (8.0 mL) [anode], and NaOPiv·H2O (2.0 equiv), HOPiv (10 equiv), MeOH (8.0 mL) [cathode] in and H-type divided cell with carbon cloth anode, nickel plate cathode, and an AMI-7001-30 membrane, constant current = 5.0 mA (Janode= 2.2 mA/cm2), ethyne balloon (1 atm), 70 °C, 3 h (2.8 F/mol). Isolated yields are shown Electrooxidative C-H/N–H [4+2] annulation with ethyne (Method B) The electrolysis was carried out in an oven-dried H-type divided cell equipped with two stir bars. 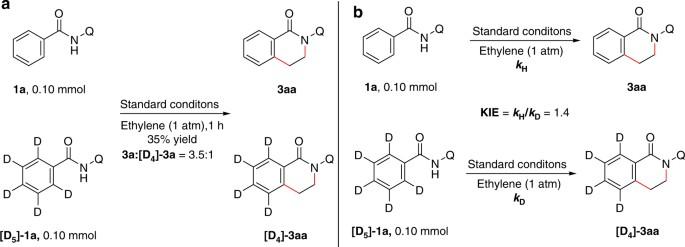Fig. 4 Kinetic isotope effect experiments.aIntermolecular competition experiment between1aand[D5]-1a.bParallel reactions with1aand[D5]-1a Carbon cloth (15 mm×15 mm×0.36 mm) was used as the anode and the nickel plate (15 mm×15 mm×1.0 mm) was used as the cathode. The two electrodes were separated by an ULTREX ® AMI-7001-30 membrane. The anodic chamber was added with amide (0.20 mmol), Co(acac) 2 (0.020 mmol, 5.1 mg), NaOPiv·H 2 O (0.40 mmol, 56.9 mg), and n Bu 4 NBF 4 (0.60 mmol, 197.6 mg) while the cathodic chamber was added with NaOPiv·H 2 O (0.40 mmol, 56.9 mg) and HOPiv (2.0 mmol, 204.3 mg). A balloon filled with ethyne (1 atm) was connected to the electrolysis system and purged for three times. Subsequently, CF 3 CH 2 OH (8.0 mL) and MeOH (8.0 mL) were added to the anodic chamber and cathodic chamber, respectively. Then electrolysis system was stirred at a constant current of 5.0 mA at 70 °C for 3 h. When the reaction was finished, the reaction mixture of the anodic chamber was washed with water and extracted with diethyl ether (10 mL × 3). The organic layers were combined, dried over Na 2 SO 4 , and concentrated. The pure product was obtained by flash column chromatography on silica gel (petroleum:ethyl acetate = 1:1). Full experimental details and characterization of the compounds are given in the Supplementary Information. 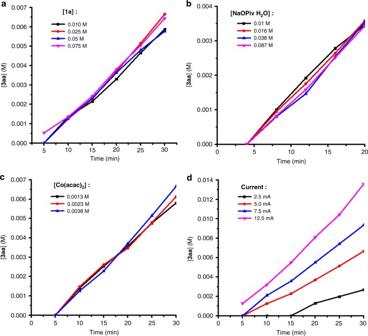Fig. 5 Kinetic studies for the cobalt-catalyzed electrooxidative C–H/N–H [4+2] annulation between 1a and ethylene.aKinetic profiles under different concentrations of1a.bKinetic profiles under different concentrations of NaOPiv·H2O.cKinetic profiles under different concentrations of Co(acac)2.dKinetic profiles under different operating currents 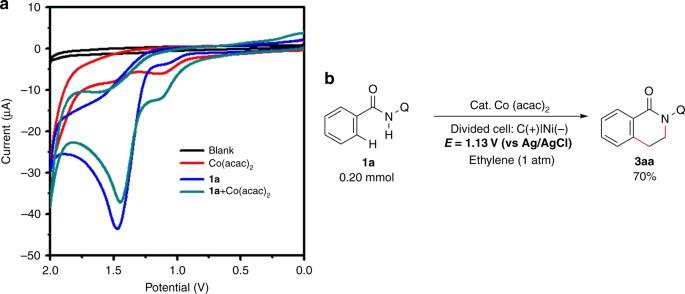Fig. 6 Study of the oxidation potential during the electrolysis.aCyclic voltammograms in CF3CH2OH (10 mL) with 0.06 MnBu4NBF4: blue line,1a(0.050 mmol); red line, Co(acac)2(0.050 mmol); green line, a mixture of Co(acac)2(0.050 mmol), and1a(0.050 mmol).bPotential controlled electrolysis at 1.13 V (vs Ag/AgCl) 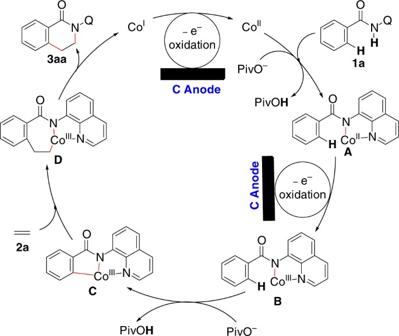Fig. 7 Proposed mechanism for the reaction between1aand2a. Tentative reaction mechanism involves anodic oxidation of the coordinated Co(II) complex to generate a Co(III) complex, intramolecular C−H activation, ethylene insertion, and reductive elimination of Co(III) species to form the annulation product, and finally a second anodic oxidation to regenerate the Co(II) catalyst Data availability The authors declare that the data supporting the findings of this study are available within the article and its Supplementary Information files.